Post-transcriptional spliceosomes are retained in nuclear speckles until splicing completion There is little quantitative information regarding how much splicing occurs co-transcriptionally in higher eukaryotes, and it remains unclear where precisely splicing occurs in the nucleus. Here we determine the global extent of co- and post-transcriptional splicing in mammalian cells, and their respective subnuclear locations, using antibodies that specifically recognize phosphorylated SF3b155 (P-SF3b155) found only in catalytically activated/active spliceosomes. Quantification of chromatin- and nucleoplasm-associated P-SF3b155 after fractionation of HeLa cell nuclei, reveals that ~80% of pre-mRNA splicing occurs co-transcriptionally. Active spliceosomes localize in situ to regions of decompacted chromatin, at the periphery of or within nuclear speckles. Immunofluorescence microscopy with anti-P-SF3b155 antibodies, coupled with transcription inhibition and a block in splicing after SF3b155 phosphorylation, indicates that post-transcriptional splicing occurs in nuclear speckles and that release of post-transcriptionally spliced mRNA from speckles is coupled to the nuclear mRNA export pathway. Our data provide new insights into when and where splicing occurs in cells. Pre-mRNA splicing is catalysed by the spliceosome, which assembles stepwise via the sequential recruitment of the U1, U2, U4, U5 and U6 small nuclear ribonucleoproteins (snRNPs) and numerous proteins to the pre-mRNA [1] . The prespliceosome is generated on interaction of U1 and U2, and the pre-catalytic B complex is subsequently formed by association of the U4/U6.U5 tri-snRNP. Conformational and compositional rearrangements, including loss of U1 and U4, lead to the activated B act complex, followed by the B* complex, which catalyses step 1 of splicing—that is, 5′-splice site (ss) cleavage and intron–3′exon lariat formation. The C complex, formed during step 1, then catalyses intron excision and ligation of the 5′ and 3′ exons (step 2). Many splicing events occur co-transcriptionally—that is, introns are removed and the neighbouring exons are spliced together while a nascent transcript is still being transcribed by RNA Pol II. The existence of co-transcriptional splicing was initially suggested by microscopy studies [2] , [3] , [4] and subsequently supported by chromatin immunoprecipitation (ChIP) analyses [5] , [6] , [7] . Evidence that splicing per se can occur co-transcriptionally has come from in situ localization (mainly by fluorescence in situ hybridization (FISH)) of transcripts from a limited number of individual endogenous or reporter genes [7] , [8] , [9] , [10] , [11] , [12] . However, some introns are excised post-transcriptionally, that is, after nascent transcripts have undergone 3′-end cleavage and subsequent release from their DNA template [13] . Introns flanking alternatively spliced exons, and those located towards the 3′ ends of pre-mRNAs, appear to be more prone to post-transcriptional splicing [4] , [9] , [14] . In Saccharomyces cerevisiae , recent high-density tilling microarray assays indicate that most yeast introns are removed co-transcriptionally [15] . Similarly, sequencing of nascent RNA transcripts revealed that most introns in D. melanogaster also undergo co-transcriptional splicing [16] . However, the global extent of co-transcriptional splicing in mammalian cells remains unclear. It is also unclear where splicing exactly occurs in the nucleus. Transcriptionally silent heterochromatin forms dense regions in the nucleus surrounded by less dense euchromatin [17] , [18] where the transcription machinery synthesizes pre-mRNA. The remaining nuclear regions, denoted the interchromatin compartment [17] , contain several nuclear bodies, including nuclear speckles (also known as interchromatin granule clusters or SC35 domains) [19] where high concentrations of spliceosome components are found. Nuclear speckles are believed to be storage sites for splicing factors [20] , and are surrounded by perichromatin fibrils where splicing is thought to occur [21] , [22] . Recent FISH studies suggest that splicing might occur directly in speckles [23] . However, as FISH does not allow the direct localization of active spliceosomes, and the RNAs followed in these studies were not generated from genes packaged in chromatin, additional data are still required to clearly elucidate the subnuclear location of co- and post-transcriptional splicing. Direct in situ investigation of the nuclear location of splicing catalysis has been hampered by the lack of tools to directly visualize active spliceosomes. Here we have developed antibodies that specifically recognize active spliceosomes, thereby enabling a global analysis of mammalian splicing in situ . By quantifying the amount of chromatin- and nucleoplasm-associated P-SF3b155 after fractionation of HeLa cell nuclei, we demonstrate that the vast majority of pre-mRNA splicing occurs co-transcriptionally. Immunofluorescence (IF) microscopy experiments with anti-P-SF3b155 antibodies, coupled with transcription inhibition and a block in splicing after phosphorylation of the SF3b155 protein, indicate that spliceosomes involved in post-transcriptional splicing accumulate in nuclear speckles. SF3b155 phosphorylation sites in active spliceosomes The U2-associated SF3b155 protein is phosphorylated during spliceosome activation and remains hyperphosphorylated until step 2 (refs 24 , 25 , 26 , 27 ). We isolated catalytically activated, human spliceosomes, and identified SF3b155 phosphorylation sites that are specific for active spliceosomes via mass spectrometry ( Fig. 1a ; Supplementary Tables S1 and S2 ). Antibodies that were highly specific for phosphorylated amino acids T211, T235, T313 or T328 of SF3b155 were subsequently generated ( Supplementary Fig. S1 ). Phospho-specific antibodies against pT313 and pT328 specifically recognized the slower migrating, phosphorylated form of SF3b155 (P-SF3b155) that formed first after 30 min of splicing in vitro ( Fig. 1b,c ; Supplementary Fig. S2 ). In contrast, antibodies recognizing a non-phosphorylated SF3b155 epitope (MC) detected SF3b155 at all time points, as well as P-SF3b155 first after 30 min ( Fig. 1b ). Western blotting of affinity-purified human B, B act and C complexes demonstrated that pT313-SF3b155 antibodies are specific for phosphorylated SF3b found solely in activated/catalytically active spliceosomes ( Fig. 1d ). 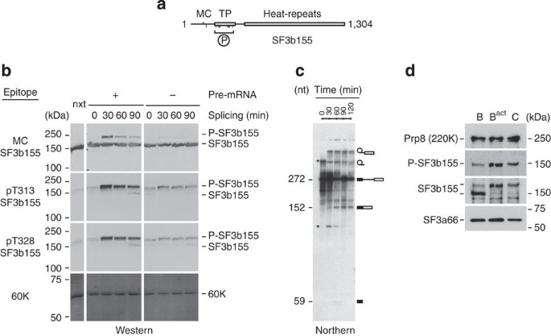Figure 1: Identification of SF3b155 amino acids phosphorylated in activated spliceosomes. (a) Schematic diagram of the U2-SF3b155 protein. TP-rich and HEAT repeats are indicated. The following SF3b155 residues were phosphorylated in affinity-purified, human Bactcomplexes: S129, T211, T235, S242, T248, S322, T326 and T328. T313 was previously identified as a target for SF3b155 phosphorylation58. Except for S129, all sites (ticks indicated by a circled P) mapped to the TP-repeat region (amino acids 207–374)24. The phosphorylation unrelated MC-epitope (amino acids 99–113) recognized by anti-SF3b155 monoclonal (MC) antibodies is indicated. (b) Characterization of anti-phospho-SF3b155 antibodies. Western blots of HeLa nuclear extract (nxt) or a time course of a splicing +/− exogenously added pre-mRNA (as indicated) were probed with antibodies specific for the MC- or phospho-T313/T328 epitopes of SF3b155. Note that the phosphorylated SF3b155 observed after 30 min in the absence of added pre-mRNA likely reflects splicing of endogenous pre-mRNAs in the extract. Loading control: 60 K protein. Panels are derived from a single blot. (c) Kinetics of pre-mRNA splicingin vitro. A reaction parallel to that inb(+ pre-mRNA) was performed and splicing after 0, 30, 60, 90 and 120 min was analysed by northern blotting using a specific probe for the pre-mRNA generated by random priming. The RNA species are indicated schematically on the left and the lengths of the pre-mRNA, spliced product and exon1 are indicated on the right in nucleotides (nt). Background signals are marked with an asterisk. (d) Affinity-purified, human B, Bactor C spliceosomal complexes were analysed by western blot with antibodies against the proteins indicated at the left. P-SF3b155 = anti-phospho-T313-SF3b155 antibodies. Note that the low level of P-SF3b155 detected in the B complex preparation is most likely due to small amounts of contaminating Bactcomplexes26. Figure 1: Identification of SF3b155 amino acids phosphorylated in activated spliceosomes. ( a ) Schematic diagram of the U2-SF3b155 protein. TP-rich and HEAT repeats are indicated. The following SF3b155 residues were phosphorylated in affinity-purified, human B act complexes: S129, T211, T235, S242, T248, S322, T326 and T328. T313 was previously identified as a target for SF3b155 phosphorylation [58] . Except for S129, all sites (ticks indicated by a circled P) mapped to the TP-repeat region (amino acids 207–374) [24] . The phosphorylation unrelated MC-epitope (amino acids 99–113) recognized by anti-SF3b155 monoclonal (MC) antibodies is indicated. ( b ) Characterization of anti-phospho-SF3b155 antibodies. Western blots of HeLa nuclear extract (nxt) or a time course of a splicing +/− exogenously added pre-mRNA (as indicated) were probed with antibodies specific for the MC- or phospho-T313/T328 epitopes of SF3b155. Note that the phosphorylated SF3b155 observed after 30 min in the absence of added pre-mRNA likely reflects splicing of endogenous pre-mRNAs in the extract. Loading control: 60 K protein. Panels are derived from a single blot. ( c ) Kinetics of pre-mRNA splicing in vitro . A reaction parallel to that in b (+ pre-mRNA) was performed and splicing after 0, 30, 60, 90 and 120 min was analysed by northern blotting using a specific probe for the pre-mRNA generated by random priming. The RNA species are indicated schematically on the left and the lengths of the pre-mRNA, spliced product and exon1 are indicated on the right in nucleotides (nt). Background signals are marked with an asterisk. ( d ) Affinity-purified, human B, B act or C spliceosomal complexes were analysed by western blot with antibodies against the proteins indicated at the left. P-SF3b155 = anti-phospho-T313-SF3b155 antibodies. Note that the low level of P-SF3b155 detected in the B complex preparation is most likely due to small amounts of contaminating B act complexes [26] . Full size image P-SF3b155 mainly associates with the chromatin fraction To test whether P-SF3b155 is associated predominantly with the transcription machinery, we fractionated HeLa cell nuclei into a soluble nucleoplasmic fraction and an insoluble fraction containing chromatin-associated material [9] . Hyperphosphorylated RPB1 (indicative of transcriptionally active RNA Pol II) was found exclusively in the chromatin fraction together with histone 3, whereas hypophosphorylated (inactive) RPB1 was nearly exclusively in the nucleoplasmic fraction ( Fig. 2a ). Thus, chromatin-associated components have not leaked into the nucleoplasmic fraction under our fractionation conditions. Most P-SF3b155 was detected in the chromatin fraction, whereas unphosphorylated SF3b155 was predominantly nucleoplasmic. Quantification of the western blot ( Supplementary Fig. S3 ) indicated that ~80 to 85% of total P-SF3b155 is associated with chromatin, whereas the remaining ~15 to 20% is nucleoplasmic. These data suggest that most active spliceosomes are associated with pre-mRNAs that are spliced co-transcriptionally, whereas 15 to 20% are associated with pre-mRNAs that undergo post-transcriptional splicing. 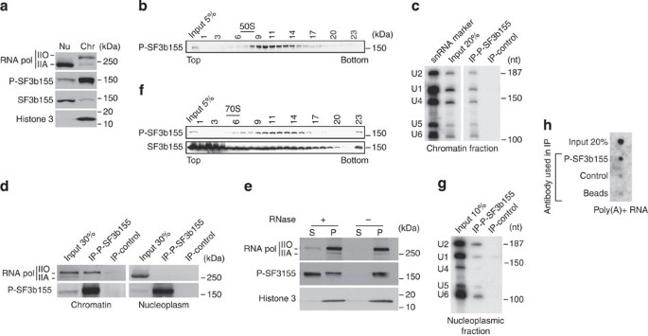Figure 2: Phosphorylated SF3b155 is found in large RNP complexes in the chromatin and nucleoplasmic fractions of HeLa cell nuclei. (a) HeLa cell nuclei were fractionated into nucleoplasmic (Nu) and chromatin (Chr) fractions as described in the Methods. Western blotting was performed with antibodies against RPB1, pT313-SF3b155, SF3b155 and histone 3. II0: phosphorylated, IIA: non-phosphorylated forms of RPB1. (b) A DSP cross-linked and sonicated chromatin fraction was subjected to 10–40% glycerol gradient centrifugation (1 h at 488,000g). Each gradient fraction was analysed by SDS–PAGE (after reversing the crosslinks), followed by western blotting with the anti-pT313-SF3b155 antibody. (c) Immunoprecipitation (IP) with anti-pT313-SF3b155 antibodies or anti-4E-T antibodies (as a control) and the sonicated chromatin fraction described in (b). The co-precipitated snRNAs and those in the input were analysed by northern blot using probes specific for U1, U2, U4, U5 and U6 snRNAs. (d) IPs with anti-pT313-SF3b155 antibodies (or control antibodies) from the chromatin and nucleoplasmic fraction were resolved by SDS–PAGE and analysed by western blot with anti-P-SF3b155, RPB1 antibodies. (f) Glycerol gradient centrifugation of untreated nucleoplasmic fraction of HeLa cells was performed as inbfor 1 h at 122,000g. Gradient fractions were analysed by western blot with anti-pT313-SF3b155 antibodies (upper panel) or those against both phosphorylated and non-phosphorylated forms of SF3b155 (lower panel). (e) The chromatin fraction was incubated with or without RNase A followed by a brief centrifugation and the supernatants (S) and pellets (P) were resolved by SDS–PAGE and analysed by western blot with anti-P-SF3b155, RPB1 and histone 3 antibodies. Equivalent amounts of the pellet and supernatant were loaded on the gel. IPs with anti-pT313-SF3b155 antibodies (or control antibodies) from nucleoplasmic fraction, co-precipitating snRNAs (g) or poly (A)+ RNA (h) were analysed by northern blot. Proportions and levels of the various snRNAs differ in the chromatin versus nucleoplasm input lanes panel c and e due to a differential distribution of snRNAs in these fractions. Figure 2: Phosphorylated SF3b155 is found in large RNP complexes in the chromatin and nucleoplasmic fractions of HeLa cell nuclei. ( a ) HeLa cell nuclei were fractionated into nucleoplasmic (Nu) and chromatin (Chr) fractions as described in the Methods. Western blotting was performed with antibodies against RPB1, pT313-SF3b155, SF3b155 and histone 3. II0: phosphorylated, IIA: non-phosphorylated forms of RPB1. ( b ) A DSP cross-linked and sonicated chromatin fraction was subjected to 10–40% glycerol gradient centrifugation (1 h at 488,000 g ). Each gradient fraction was analysed by SDS–PAGE (after reversing the crosslinks), followed by western blotting with the anti-pT313-SF3b155 antibody. ( c ) Immunoprecipitation (IP) with anti-pT313-SF3b155 antibodies or anti-4E-T antibodies (as a control) and the sonicated chromatin fraction described in ( b ). The co-precipitated snRNAs and those in the input were analysed by northern blot using probes specific for U1, U2, U4, U5 and U6 snRNAs. ( d ) IPs with anti-pT313-SF3b155 antibodies (or control antibodies) from the chromatin and nucleoplasmic fraction were resolved by SDS–PAGE and analysed by western blot with anti-P-SF3b155, RPB1 antibodies. ( f ) Glycerol gradient centrifugation of untreated nucleoplasmic fraction of HeLa cells was performed as in b for 1 h at 122,000 g . Gradient fractions were analysed by western blot with anti-pT313-SF3b155 antibodies (upper panel) or those against both phosphorylated and non-phosphorylated forms of SF3b155 (lower panel). ( e ) The chromatin fraction was incubated with or without RNase A followed by a brief centrifugation and the supernatants (S) and pellets (P) were resolved by SDS–PAGE and analysed by western blot with anti-P-SF3b155, RPB1 and histone 3 antibodies. Equivalent amounts of the pellet and supernatant were loaded on the gel. IPs with anti-pT313-SF3b155 antibodies (or control antibodies) from nucleoplasmic fraction, co-precipitating snRNAs ( g ) or poly (A)+ RNA ( h ) were analysed by northern blot. Proportions and levels of the various snRNAs differ in the chromatin versus nucleoplasm input lanes panel c and e due to a differential distribution of snRNAs in these fractions. Full size image Next, we assayed via gradient sedimentation and immunoprecipitation (IP) studies whether the P-SF3b155 in the chromatin and nucleoplasmic fractions is incorporated into spliceosomes. Spliceosomes formed on single-intron pre-mRNAs in vitro have sedimentation coefficients up to ~45–50S (ref. 28 ). The chromatin fraction was completely solubilized via sonication after first preserving the integrity of spliceosomes by crosslinking with dithiobis-(succinimidylpropionate) (DSP), a homobifunctional crosslinker that stabilizes protein–protein interactions; a similar strategy was successfully used to analyse other chromatin-associated complexes [29] . Nearly, all P-SF3b155 in the chromatin fraction was present in complexes sedimenting faster than 50S on glycerol gradients ( Fig. 2b ). IP of the peak gradient fractions followed by northern blotting revealed that the U1, U2, U4, U5 and U6 spliceosomal snRNAs co-precipitate together with P-SF3b155 ( Fig. 2c ). Although active spliceosomes formed in vitro consist of U2, U5 and U6 snRNAs [26] , the presence of U1 and U4 may be due to the co-IP of newly assembling/non-activated spliceosomes formed on introns neighbouring those containing active spliceosomes. IP of the chromatin fraction after mild shearing (instead of crosslinking followed by sonication), to release active spliceosomes while preserving their association with the polymerase, revealed that solely the hyperphosphorylated form of RPB1 co-precipitated with P-SF3b155 ( Fig. 2d ). Importantly, RNase A treatment led to the release of P-SF3b155 from the chromatin fraction ( Fig. 2e ), indicating that association of active spliceosomes with chromatin is RNA dependent. Taken together, these data support the idea that chromatin-associated P-SF3b155 is present in active spliceosomes engaged in co-transcriptional splicing. When the nucleoplasmic fraction, which was analysed without prior crosslinking and sonication, was subjected to glycerol gradient centrifugation, essentially all P-SF3b155 was detected in complexes with S-values >70S ( Fig. 2f ), whereas large amounts of non-phosphorylated SF3b155 were found at the top of the gradient. Thus, P-SF3b155 does not exist as part of 17S U2 snRNPs or free SF3b complexes in the nucleoplasm. Nucleoplasmic P-SF3b155 was mainly associated with U2, U5 and U6 snRNAs, when compared with the input signals ( Fig. 2g ), consistent with its presence in B act or later spliceosomal complexes. Furthermore, no RPB1 ( Fig. 2f ), but ~6.5% of the poly(A)+ RNA (from soluble cytoplasmic and nucleoplasmic fractions prepared as described in Supplementary Fig. S3 ), was co-precipitated together with P-SF3b155 ( Fig. 2h ), consistent with nucleoplasmic P-SF3b155 associating with active spliceosomes engaged in post-transcriptional splicing. Detection of splicing-dependent SF3b155 phosphorylation in situ To investigate where splicing occurs in cells, we performed IF microscopy with anti-pT313-SF3b155 antibodies. Exclusively nuclear staining of HeLa cells, with clear exclusion of the nucleoli was observed ( Fig. 3a ). Significantly, inhibition of transcription (and thus the supply of pre-mRNA) with 5,6-dichloro-1-β- d -ribofuranosylbenzimidazole (DRB), confirmed by the loss of the IF signal of antibodies specific for Ser5 phosphorylation of the CTD heptad repeat of RNA Pol II (ref. 30 ), nearly abolished the anti-P-SF3b155 signal ( Fig. 3b ). In contrast, the signal obtained with antibody recognizing all forms of SF3b155 changed only minimally. Inhibition of splicing directly with spliceostatin A (SSA), which leads to the formation of non-functional prespliceosomes [31] , [32] also severely reduced the P-SF3b155 signal ( Fig. 3c ). In SSA-treated cells, nuclear speckles appeared as more rounded dots compared with control cells ( Fig. 3c ), as shown by the distribution of the spliceosomal protein SC35, a typical nuclear speckle marker [33] ; however, the overall intensity of the SC35 signal was unaffected. Collectively, these experiments provide evidence that the IF signal observed in situ with our anti-P-SF3b155 antibodies corresponds to active spliceosomes. 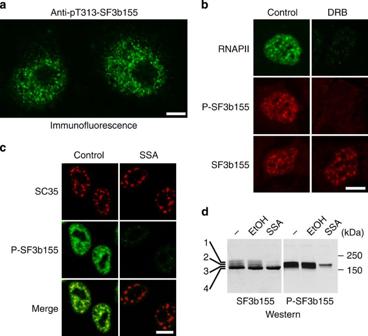Figure 3: Anti-P-SF3b155 immunofluorescence (IF) signal is dependent on ongoing transcription and splicing. (a) HeLa cells were stained with the anti-pT313-SF3b155 antibody (green) and visualized by IF microscopy. (b) Cells treated with DRB for 3.5 h were analysed by double IF microscopy using anti-pT313-SF3b155 (green) and antibodies against elongating RNA polymerase II (RNAPII, red) or the monoclonal (MC)-epitope of SF3b155 (MC antibody, red). (c) Double IF microscopy of cells treated with spliceostatin A (SSA) for 2 h using anti-SC35 (red) and anti-pT313-SF3b155 (green) antibodies. (d) Western blot of proteins isolated from SSA-treated or control cells (−, EtOH), performed with the indicated antibodies. Scale bars, 10 μm. Figure 3: Anti-P-SF3b155 immunofluorescence (IF) signal is dependent on ongoing transcription and splicing. ( a ) HeLa cells were stained with the anti-pT313-SF3b155 antibody (green) and visualized by IF microscopy. ( b ) Cells treated with DRB for 3.5 h were analysed by double IF microscopy using anti-pT313-SF3b155 (green) and antibodies against elongating RNA polymerase II (RNAPII, red) or the monoclonal (MC)-epitope of SF3b155 (MC antibody, red). ( c ) Double IF microscopy of cells treated with spliceostatin A (SSA) for 2 h using anti-SC35 (red) and anti-pT313-SF3b155 (green) antibodies. ( d ) Western blot of proteins isolated from SSA-treated or control cells (−, EtOH), performed with the indicated antibodies. Scale bars, 10 μm. Full size image We also assayed the phosphorylation status of SF3b155 in control versus SSA-treated cells by western blotting ( Fig. 3d ). A dramatic reduction in phosphorylated SF3b155 species upon SSA treatment was observed with both anti-SF3b155 (MC-specific) and anti-pT313-SF3b155 antibodies. Comparison of the two blots allowed us to unequivocally assign the upper two bands to splicing-related phosphorylation of SF3b155 occurring in cells. Quantification of the intensities of the four SF3b bands detected with the MC-specific antibody revealed that ~13–16% of SF3b155 is phosphorylated in vivo and—by inference—engaged in active splicing. Subnuclear localization of active spliceosomes We next performed IF microscopy with a cell line that stably expresses histone 2B fused to GFP (H2B-GFP) [34] , to determine the relative spatial organization of chromatin, speckles and active spliceosomes. Consistent with previous observations [17] , chromatin (H2B: blue) was non-uniformly distributed in the nucleus, with intense IFe (indicating dense chromatin) alternating with less intense regions ( Fig. 4a ). Nuclear speckles (SC35: red) almost always fit snugly into the less dense 'holes' seen in the chromatin ( Fig. 4a , SC35/H2B merge). Active spliceosomes visualized with anti-pT313-SF3b155 antibodies (P-SF3b155: green) adopted a web-like structure throughout the nucleus, and were nearly exclusively detected in the less dense chromatin areas ( Fig. 4a ). Strikingly, a large portion of P-SF3b155 accumulated in the vicinity of speckles ( Fig. 4a–c ). A close examination of z-stack sections revealed that most of the P-SF3b155 signal surrounds the SC35-containing regions ( Fig. 4d ). However, in the z-sections that cut through the speckle, an overlap between the P-SF3b155 and SC35 signals was readily observable. Analyses of deconvolved z-stack pictures with a co-localization analysis software [35] (JACOP, image J), indicated that 9–25% of total P-SF3b155 co-localized with SC35, whereas 90% of SC35 co-localized with P-SF3b155 (as determined by Manders' coefficients). Thus, active spliceosomes not only localize to the speckle periphery but also are found within speckles. 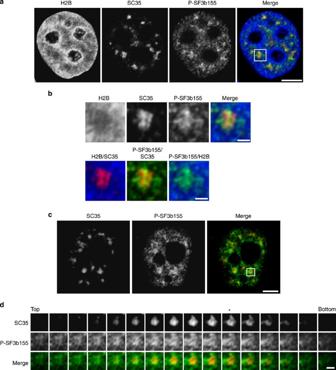Figure 4: Active spliceosomes localize to the periphery of nuclear speckles and are excluded from dense chromatin. (a) Triple immunofluorescence (IF) microscopy of HeLa cells expressing Histone 2B-GFP (blue). Speckles were visualized with the anti-SC35 antibody (red) and active spliceosomes with the anti-pT313-SF3b155 antibody (green). Scale bar, 5 μm. (b) Magnification of the boxed region ina. All possible two-way overlays are shown. (c) Speckles were visualized with anti-SC35 antibody (red), and active spliceosomes with the anti-pT313-SF3b155 antibody (green). (d) Magnification of the boxed region inc. Z-Stack sections were acquired (optical section of 400–500 nm) and deconvolved. All optical sections from the z-stack are shown from top to bottom. The star indicates the optical section shown inc. Scale bar, 1 μm. Figure 4: Active spliceosomes localize to the periphery of nuclear speckles and are excluded from dense chromatin. ( a ) Triple immunofluorescence (IF) microscopy of HeLa cells expressing Histone 2B-GFP (blue). Speckles were visualized with the anti-SC35 antibody (red) and active spliceosomes with the anti-pT313-SF3b155 antibody (green). Scale bar, 5 μm. ( b ) Magnification of the boxed region in a . All possible two-way overlays are shown. ( c ) Speckles were visualized with anti-SC35 antibody (red), and active spliceosomes with the anti-pT313-SF3b155 antibody (green). ( d ) Magnification of the boxed region in c . Z-Stack sections were acquired (optical section of 400–500 nm) and deconvolved. All optical sections from the z-stack are shown from top to bottom. The star indicates the optical section shown in c . Scale bar, 1 μm. Full size image Post-transcriptional spliceosomes localize to speckles To distinguish between active spliceosomes involved in co- versus post-transcriptional splicing, we first stalled the splicing reaction after B complex formation, which should enrich for active spliceosomes and lead to enhanced accumulation of post-transcriptional spliceosomes. Thus, we performed RNA interference (RNAi)-mediated knockdown of the spliceosomal protein CDC5L, a component of the human Prp19 complex. Previous studies indicated that in humans CDC5L is required for splicing, at least in vitro , at a stage after B complex formation, before step 2 of splicing [36] , [37] , but the precise step at which it acts is not clear. Approximately 80% of CDC5L was depleted 60 h after short interfering RNA (siRNA) transfection ( Fig. 5a , full blots shown in Supplementary Fig. S4 ), and correspondingly, a strong reduction in the CDC5L IF signal was observed in ΔCDC5L cells ( Fig. 5b ), confirming the efficacy of the knockdown. Importantly, no significant loss of P-SF3b155 on knockdown of CDC5L was detected by IF microscopy ( Fig. 5d ) or immunoblotting ( Fig. 5a ). Indeed, a general increase in both P-SF3b155 and poly(A)+ RNA (visualized by FISH) in ΔCDC5L cells was observed ( Fig. 5d ), consistent with the accumulation of post-transcriptional spliceosomes due to splicing inhibition. In contrast, knockdown of the splicing factor Prp8 (required for B complex formation) led to a clear reduction in P-SF3b155 signal ( Supplementary Fig. S5 ). Thus, CDC5L knockdown appears to block splicing at a step after SF3b155 phosphorylation. 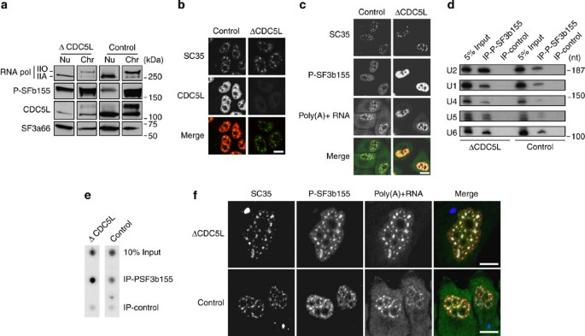Figure 5: Stalled spliceosomes accumulate within speckles in CDC5L-depleted cells. (a) Nuclei of control cells or those depleted of CDC5L by RNAi (ΔCDC5L) were fractionated into nucleoplasmic (Nu) and chromatin (Chr) fractions. (a) Identical amounts of each fraction were resolved by SDS–PAGE and analysed by western blot with antibodies against RNA polymerase II large subunit RPB1, P-SF3b155, CDC5L or SF3a66 (loading control). Panels are derived from a single blot with the same exposure time. Note that CDC5L knockdown also led to a reduction in active transcription, as evidenced by the reduced levels of phosphorylated RPB1. (b) Double immunofluorescence microscopy with control and ΔCDC5L cells: SC35 (green) and CDC5L (red). Individual channels are shown in black and white and the merged channels in colour. (c) Identical cells were stained with anti-SC35 (blue) and anti-pT313-SF3b155 (red) antibodies, and poly(A)+ RNA was visualized by FISH with a fluorescently labelled oligo-d(T) probe (green). Note that the immunofluorescence signals are not quantitative, as the P-SF3b155 signal in the ΔCDC5L cells is not in the dynamic range. (d) Immunoprecipitation (IP) with control or anti-pT313-SF3b antibodies and the nucleoplasmic fractions of ΔCDC5L and control cells. Co-precipitated RNAs were analysed by denaturing PAGE followed by northern blot with32P-labelled probes specific for the indicated snRNA. (e) Dot blot of RNA co-precipitated with the indicated antibodies and probed with32P-oligo dT. (f) Projection of the maximum intensities of stacks recorded from bottom to the top of control and ΔCDC5L cells. SC35, P-SF3b155 and poly(A)+ RNA were visualized as inc. Scale bars, 10 μm. Figure 5: Stalled spliceosomes accumulate within speckles in CDC5L-depleted cells. ( a ) Nuclei of control cells or those depleted of CDC5L by RNAi (ΔCDC5L) were fractionated into nucleoplasmic (Nu) and chromatin (Chr) fractions. ( a ) Identical amounts of each fraction were resolved by SDS–PAGE and analysed by western blot with antibodies against RNA polymerase II large subunit RPB1, P-SF3b155, CDC5L or SF3a66 (loading control). Panels are derived from a single blot with the same exposure time. Note that CDC5L knockdown also led to a reduction in active transcription, as evidenced by the reduced levels of phosphorylated RPB1. ( b ) Double immunofluorescence microscopy with control and ΔCDC5L cells: SC35 (green) and CDC5L (red). Individual channels are shown in black and white and the merged channels in colour. ( c ) Identical cells were stained with anti-SC35 (blue) and anti-pT313-SF3b155 (red) antibodies, and poly(A)+ RNA was visualized by FISH with a fluorescently labelled oligo-d(T) probe (green). Note that the immunofluorescence signals are not quantitative, as the P-SF3b155 signal in the ΔCDC5L cells is not in the dynamic range. ( d ) Immunoprecipitation (IP) with control or anti-pT313-SF3b antibodies and the nucleoplasmic fractions of ΔCDC5L and control cells. Co-precipitated RNAs were analysed by denaturing PAGE followed by northern blot with 32 P-labelled probes specific for the indicated snRNA. ( e ) Dot blot of RNA co-precipitated with the indicated antibodies and probed with 32 P-oligo dT. ( f ) Projection of the maximum intensities of stacks recorded from bottom to the top of control and ΔCDC5L cells. SC35, P-SF3b155 and poly(A)+ RNA were visualized as in c . Scale bars, 10 μm. Full size image In ΔCDC5L cells, an approximately threefold increase in nucleoplasmic P-SF3b155, relative to the control, was observed ( Fig. 5a ), whereas the amount of chromatin-associated P-SF3b155 was essentially unchanged. Furthermore, ~3 times more spliceosomal U1-U6 snRNAs (in particular U2, U5 and U6), and ~2.5 times more poly(A)+ RNA were co-precipitated together with P-SF3b155 from the nucleoplasmic fractions of ΔCDC5L versus control cells ( Fig. 5d,e ). This suggests that on CDC5L knockdown, P-SF3b155 in the nucleoplasm is still associated with spliceosomes stalled on polyadenylated pre-mRNAs. A closer examination of the IF pictures revealed clear overlap of SC35, P-SF3b155 and poly(A)+ RNA in ΔCDC5L cells ( Fig. 5f ), suggesting that pre-mRNA transcripts associated with stalled spliceosomes accumulate in speckles. Although poly(A)+ RNAs reside in speckles under normal conditions [22] ( Supplementary Fig. S6 ), in ΔCDC5L cells there was enhanced accumulation of poly(A)+ RNA in these structures, consistent with a block in splicing. Taken together, these data indicate that CDC5L knockdown leads to the accumulation of post-transcriptional spliceosomes in the nucleoplasm. To abolish co-transcriptional splicing, we blocked transcription with DRB. P-SF3b155 was dramatically reduced in the nucleoplasmic and the chromatin fraction of control knockdown cells treated with DRB for 3.5 h ( Fig. 6a ). In ΔCDC5L cells, DRB treatment led to a strong reduction in chromatin-associated P-SF3b155, whereas the amount of P-SF3b155 in the nucleoplasmic fraction was identical to that in dimethylsulphoxide (DMSO)-treated ΔCDC5L cells ( Fig. 6a ). Thus, the amount of active spliceosomes associated with chromatin is severely reduced in ΔCDC5L cells on transcription inhibition. 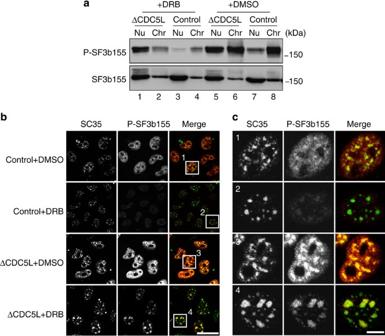Figure 6: Post-transcriptional spliceosomes localize to nuclear speckles. (a) HeLa cells were incubated with a control siRNA (control) or CDC5L siRNA (ΔCDC5L) for 60 h and then treated with DMSO (as a control; lanes 5–8) or the transcription inhibitor DRB (lanes 1–4) for 210 min. Equivalent amounts of nucleoplasmic (Nu) and chromatin (Chr) fractions were analysed in each lane by western blot with anti-P-SF3b155 and anti-SF3b155 antibodies. (b) Identical cells as described inawere analysed by immunofluorescence microscopy with anti-SC35 antibodies as a speckle marker (green) and anti-P-SF3b155 antibodies to visualize active spliceosomes (red). Individual channels are shown in black and white and the merged channels in colour. The same microscope settings were used to record all images. Scale bar, 50 μm. (c) Magnification of a single cell corresponding to the boxed area shown in the merge panel inb. Figure 6: Post-transcriptional spliceosomes localize to nuclear speckles. ( a ) HeLa cells were incubated with a control siRNA (control) or CDC5L siRNA (ΔCDC5L) for 60 h and then treated with DMSO (as a control; lanes 5–8) or the transcription inhibitor DRB (lanes 1–4) for 210 min. Equivalent amounts of nucleoplasmic (Nu) and chromatin (Chr) fractions were analysed in each lane by western blot with anti-P-SF3b155 and anti-SF3b155 antibodies. ( b ) Identical cells as described in a were analysed by immunofluorescence microscopy with anti-SC35 antibodies as a speckle marker (green) and anti-P-SF3b155 antibodies to visualize active spliceosomes (red). Individual channels are shown in black and white and the merged channels in colour. The same microscope settings were used to record all images. Scale bar, 50 μm. ( c ) Magnification of a single cell corresponding to the boxed area shown in the merge panel in b . Full size image DRB treatment abolished the P-SF3b155 signal in control knockdown cells ( Fig. 6b,c ). In ΔCDC5L cells treated with DRB (but not DMSO), P-SF3b155 appeared to localize almost exclusively within nuclear speckles ( Fig. 6c ). A close examination of Z-stack sections confirmed that P-SF3b155 is distributed evenly throughout the whole speckle ( Supplementary Fig. S7 ), indicating that post-transcriptional spliceosomes stalled before step 1 of splicing accumulate in speckles. Retention of post-transcriptional spliceosomes in speckles We wished to determine whether the stalled spliceosomes that occur after RNAi-mediated knockdown of CDC5L for 48 h (which also led to P-SF3b155 accumulation within speckles, Supplementary Fig. S8 ) and localize in speckles are still functionally competent, as opposed to dead-end complexes. To address this cells were transfected with a plasmid-encoding GFP-CDC5L, cultured for 12 h post transfection, and then analysed by IF microscopy. Transfection of GFP-CDC5L had little effect on the intensity and distribution of the P-SF3b155 or poly(A)+ RNA signals in control cells ( Fig. 7a,c ). In contrast, expression of GFP-CDC5L in ΔCDC5L cells resulted in a strong reduction in the overall P-SF3b155 signal in ~75% of all cells examined ( n =104), and a milder, yet significant reduction in ~15% of the cells. Closer examination of ΔCDC5L cells showed that GFP-CDC5L expression restored the P-SF3b155 distribution to that observed in control cells; that is, P-SF3b155 no longer accumulated within speckles ( Fig. 7b ). For comparison, in neighbouring cells that had not been transfected, a strong accumulation of P-SF3b155 within speckles was still observed ( Fig. 7a,b ). In ΔCDC5L cells that did not express CDC5L-GFP, P-SF3b155 accumulated in speckles together with poly(A)+ RNA ( Fig. 7c,d ). In contrast, in ~78% of the ΔCDC5L cells expressing GFP-CDC5L ( n =110), the amount of poly(A)+ RNA within speckles was reduced to a level comparable to that of control cells ( Fig. 7d ). This effect was specific for GFP-CDC5L, as expression of the GFP-SmD1 protein did not affect the distribution of either P-SF3b155 or poly(A)+RNA ( Supplementary Fig. S9 ). Notably, in all cells examined, the decrease in poly(A)+ RNA signal correlated with a decrease in the P-SF3b155 signal. 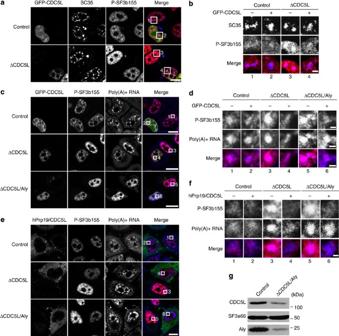Figure 7: Addition of CDC5L to ΔCDC5L cells abolishes accumulation of P-SF3b155 and Poly(A)+ RNA in speckles. (a) Cells depleted of CDC5L by RNAi (ΔCDC5L) or control cells were transfected with GFP-CDC5L 48 h post-siRNA transfection and cultured for an additional 12 h. Immunofluorescence microscopy was performed with anti-SC35 antibodies (as a speckle marker) (blue) and anti-P-SF3b155 antibodies (red). GFP-CDC5L is shown in green. (b) Magnification of speckles corresponding to the framed areas shown ina. Frames 1 and 3 are from cells not expressing GFP-CDC5L, 2 and 4 from GFP-CDC5L-transfected cells. (c) Immunofluorescence microscopy of cells depleted of CDC5L (ΔCDC5L) or CDC5L and Aly (ΔCDC5L/Aly) by RNAi. Poly(A)+ RNA was visualized by FISH and active spliceosomes by anti-P-SF3b155 antibodies. Each channel is shown individually in black and white and then merged. GFP-CDC5L is displayed in green, P-SF3b155 in red and Poly(A)+ RNA in blue. (d) Magnification of speckles corresponding to the framed areas shown inc. Frames are as described inb. (e) Cells depleted of CDC5L (ΔCDC5L) or CDC5L and Aly (ΔCDC5L/Aly) by RNAi or control cells were microinjected with purified Prp19/CDC5L complexes, plus FITC-labelled dextran (green) as tracer, 60 h post-siRNA transfection and cultured for 45 min. Immunofluorescence microscopy was performed as incandd. (f) Magnification of speckles corresponding to the framed areas shown ine. (g) Total extract from ΔCDC5L or ΔCDC5L/Aly cells was analysed by western blot using antibodies against CDC5L, Aly or SF3a66 (as a loading control). Scale bar, 10 μm. Figure 7: Addition of CDC5L to ΔCDC5L cells abolishes accumulation of P-SF3b155 and Poly(A)+ RNA in speckles. ( a ) Cells depleted of CDC5L by RNAi (ΔCDC5L) or control cells were transfected with GFP-CDC5L 48 h post-siRNA transfection and cultured for an additional 12 h. Immunofluorescence microscopy was performed with anti-SC35 antibodies (as a speckle marker) (blue) and anti-P-SF3b155 antibodies (red). GFP-CDC5L is shown in green. ( b ) Magnification of speckles corresponding to the framed areas shown in a . Frames 1 and 3 are from cells not expressing GFP-CDC5L, 2 and 4 from GFP-CDC5L-transfected cells. ( c ) Immunofluorescence microscopy of cells depleted of CDC5L (ΔCDC5L) or CDC5L and Aly (ΔCDC5L/Aly) by RNAi. Poly(A)+ RNA was visualized by FISH and active spliceosomes by anti-P-SF3b155 antibodies. Each channel is shown individually in black and white and then merged. GFP-CDC5L is displayed in green, P-SF3b155 in red and Poly(A)+ RNA in blue. ( d ) Magnification of speckles corresponding to the framed areas shown in c . Frames are as described in b . ( e ) Cells depleted of CDC5L (ΔCDC5L) or CDC5L and Aly (ΔCDC5L/Aly) by RNAi or control cells were microinjected with purified Prp19/CDC5L complexes, plus FITC-labelled dextran (green) as tracer, 60 h post-siRNA transfection and cultured for 45 min. Immunofluorescence microscopy was performed as in c and d . ( f ) Magnification of speckles corresponding to the framed areas shown in e . ( g ) Total extract from ΔCDC5L or ΔCDC5L/Aly cells was analysed by western blot using antibodies against CDC5L, Aly or SF3a66 (as a loading control). Scale bar, 10 μm. Full size image We also microinjected purified human hPrp19/CDC5L complexes directly into the cytoplasm of ΔCDC5L cells 60 h after siRNA transfection. After 45 min, a strong reduction in the P-SF3b155 and poly(A)+ RNA signals in speckles, was observed in the microinjected cells ( Fig. 7e,f ), consistent with a 0.4–7 min half time for splicing in mammalian cells [38] . These results support the idea that add-back of CDC5L to ΔCDC5L cells allows stalled spliceosomes to complete splicing, leading to a decrease in P-SF3b155, and that the resulting post-transcriptionally spliced mRNAs are subsequently released from speckles. Release of spliced mRNA from speckles is coupled to mRNA export We next tested whether release of poly(A)+ RNA from speckles induced by CDC5L complementation is coupled to its export to the cytoplasm, by additionally blocking mRNA export via knockdown of the export essential factor Aly [23] . RNAi-mediated knockdown of both CDC5L and Aly led to a ~75% and ~90% reduction in each protein, respectively, after 48 h ( Fig. 7g ). In ΔCDC5L/Aly cells transfected with GFP-CDC5L and analysed after 12 h (that is, 60 h post-siRNA transfection), there was a marked decrease in P-SF3b155 in speckles compared with non-transfected ΔCDC5L/Aly cells ( Fig. 7c,d ). However, no decrease in poly(A)+ RNA in speckles was observed between transfected and non-transfected ΔCDC5L/Aly cells ( Fig. 7c,d ), indicating that the block in mRNA export prevents the spliced mRNAs from leaving the speckles. Identical results were obtained by microinjecting purified hPrp19/CDC5L complexes into ΔCDC5L/Aly cells ( Fig. 7e,f ). Thus, after post-transcriptional splicing in speckles is completed, release of the resultant mRNAs is coupled to the nuclear mRNA export pathway. Thus, it is highly likely that most of the released mRNAs are transported to the cytoplasm, as opposed to being dead-end products that are simply degraded. We have generated antibodies specific for phosphorylation events occurring solely in activated/catalytically active spliceosomes, allowing for the first time a global analysis of when (relative to transcription) and where in the nucleus of mammalian cells active splicing occurs. Our SF3b155 phosphorylation-specific antibodies are well-suited for detecting activated/active spliceosomes both in vitro and in situ as demonstrated by their specificity in western blots for splicing-dependent P-SF3b155 species both in vitro ( Fig. 1 ) and in cells ( Fig. 3 ), as well as by their ability to immunoprecipitate RNP complexes containing primarily U2, U5 and U6 snRNPs, and poly(A)+ RNA, from the nucleoplasmic fraction of HeLa nuclei ( Fig. 2 ). In addition, the IF signal of P-SF3b155 in HeLa cell nuclei was dependent on ongoing transcription and splicing ( Fig. 3 ) and localized primarily in nuclear regions, where co-transcriptional splicing catalysis is expected to occur—that is, in regions of decompacted chromatin and at the periphery of nuclear speckles ( Fig. 4 ). As these antibodies detect active spliceosomes independent of the pre-mRNA substrate, they represent a unique tool to dissect splicing in live cells on a global level. Indeed, previous analyses of pre-mRNA splicing in mammalian cells were limited to individual pre-mRNA species or small subsets of pre-mRNAs, and were followed in situ by FISH, ChIP or, after nuclear fractionation, by RT–PCR [7] , [9] , [39] . The fate of a handful of pre-mRNAs was followed by microinjection of a reporter gene or transcript [23] , [40] , [41] , [42] , which might not reflect the same fate as that of nascent transcripts transcribed from chromatin-associated genes. Thus, an added advantage of our antibodies is that they allow us to follow the fate of pre-mRNAs that are transcribed and spliced under physiological conditions. Our data indicate that 80 to 85% of active spliceosomes are associated with pre-mRNAs that are in the process of being transcribed (that is, co-transcriptional spliceosomes), whereas 15 to 20% are associated with pre-mRNAs that have undergone 3′-end cleavage and subsequent release from their DNA template into the nucleoplasm (that is, post-transcriptional spliceosomes). The reliability of these numbers is dependent on several factors such as the efficiency with which we can separate the chromatin and nucleoplasmic fractions of HeLa cell nuclei, and the assumption that after polyadenylation and cleavage, partially unspliced transcripts no longer associate with chromatin. That chromatin-associated components do not leak into the soluble nucleoplasmic fraction was supported by western blot analyses ( Fig. 2 ). Several previous reports suggested that nascent transcripts that are unable to be processed are retained at sites of transcription [39] , [43] , [44] . However, this retention was only observed when U1 and/or U2 snRNPs were prevented from associating with the newly transcribed pre-mRNA [39] , [43] , which is not the case when we block splicing either with SSA or by knockdown of CDC5L [39] . That there are at most only low levels of contaminating post-transcriptional spliceosomes in our chromatin fraction is supported by the fact that under conditions where we expect little or no co-transcriptional splicing, but rather post-transcriptional splicing (that is, after inhibiting transcription with DRB and splicing with SSA) there are only low levels (~15% of the amount found in control cells) of spliceosomes containing P-SF3b155 in the chromatin fraction ( Fig. 6a , cf lanes 2, 4 and 8), which translates into ~12% of the total P-SF3b155 signal. As transcription did not appear to be 100% inhibited (based on the IF signal of hyperphosphorylated RPB1, Fig. 3b ), some of this residual P-SF3b155 may also come from the low level of transcription taking place even after DRB treatment. Significantly, on CDC5L knockdown alone, which leads to an increase in post-transcriptional spliceosomes, there is no increase in the P-SF3b155 signal in the chromatin fraction of knockdown cells, which should occur if the chromatin fraction were in fact heavily contaminated with post-transcriptional spliceosomes. Thus, maximally, there could potentially be ~12% less co-transcriptional splicing and ~12% more post-transcriptional splicing than calculated, which would still mean that at least ~70% of splicing occurs co-transcriptionally in mammalian cells. The percent of co- and post-transcriptional splicing that we have quantified is also consistent with our IF data, showing that the majority of the P-SF3b155 signal (80–90%) does not localize to nuclear speckles where, based on our data post-transcriptional splicing appears to occur, but rather to subnuclear regions where active transcription takes place. Finally, recent studies also indicate that the majority of splicing events occur co-transcriptionally both in yeast and fruit flies [15] , [16] . As in the current study, we have not identified which RNA species co-IP with P-SF3b155 in the chromatin versus nucleoplasmic fractions, we cannot rule out that there is a differential distribution of highly expressed versus less abundant RNA species in these fractions. Likewise, the nuclear distribution of low abundance transcripts associated with P-SF3b155 may escape detection via IF microscopy due to the weak intensity of their IF signal. Post-transcriptional splicing, where transcription and splicing are uncoupled, appears in part to arise due to the slower kinetics of splicing relative to transcription [13] . Indeed, pre-mRNA introns located at the 3′ end of multiple intron transcripts are more frequently spliced post-transcriptionally, presumably because transcription termination and cleavage at the polyadenylation site occur before the splicing machinery manages to catalyse their removal [4] , [9] . Consistent with this idea, we could alter the ratio between co- and post-transcriptional splicing in favour of the latter by slowing down and/or blocking splicing via knockdown of the splicing essential factor CDC5L. In higher eukaryotes, where alternative splicing is prevalent, some alternative splicing events occur primarily post-transcriptionally, even when the splicing of neighbouring introns occurs co-transcriptionally [9] , [14] . However, it is presently unclear how widespread post-transcriptional splicing of alternatively spliced exons is. Thus, it will be interesting in the future to determine which constitutive and which alternative splicing events occur post-transcriptionally (and to what extent), by assaying the nature of the RNAs associated with active spliceosomes in the nucleoplasmic fraction of HeLa cell nuclei by performing quantitative microarray profiling. We observed a strong accumulation of both P-SF3b155 and poly(A)+ RNA in nuclear speckles on blocking transcription and splicing (by CDC5L knockdown) subsequent to SF3b155 phosphorylation ( Fig. 6 ), and this enhanced accumulation was reversed when the block in splicing was alleviated by expression of GFP-CDC5L or microinjection of hPrp19/CDC5L complexes ( Fig. 7 ). Our data indicate that most polyadenylated pre-mRNAs that have not completed splicing, and thus remain associated with spliceosomes, accumulate in speckles where they appear to be retained until completion of their splicing. These data thus suggest a new role for speckles, namely as sites involved in post-transcriptional splicing. Indeed, in untreated HeLa cells, ~10% of active spliceosomes (that is, P-SF3b155 signal) co-localized with the speckle marker SC35 ( Fig. 5 ), indicating they are present in speckles under normal conditions. As transcription does not appear to take place in speckles [45] , [46] , it is likely that the P-SF3b155 in speckles in untreated HeLa cells is also engaged in post-transcriptional splicing. However, we cannot exclude that post-transcriptional splicing may additionally or alternatively occur elsewhere in the nucleus. That speckles might serve not only as storage sites for splicing factors but also as sites for splicing per se , was suggested by previous studies [23] , [24] , [41] , [42] . Retention of spliceosomes (and their pre-mRNA substrate) in speckles could be due to the fact that all splicing factors are thought to possess their own speckle localization signal; thus spliceosomes, which are composed of a multitude of splicing factors, might have a high affinity for speckles [20] . This in turn would suggest that spliced mRNAs (which no longer associate with numerous splicing factors) would no longer be retained in speckles. However, our data indicate that the release of post-transcriptionally spliced mRNAs from speckles is actively dependent on the mRNA nuclear export pathway. That is, when both the export pathway, by knockdown of the export factor Aly, and splicing (via CDC5L knockdown) were blocked, poly(A)+RNA stayed in speckles even when splicing activity was subsequently restored by adding back CDC5L ( Fig. 7 ). Thus, spliceosome disassembly after the completion of splicing is not sufficient for the release of spliced mRNA from speckles. The localization of post-transcriptional spliceosomes within speckles, where the concentration of splicing factors is the highest in the nucleus, might have a profound influence on the outcome of alternative splicing. As we can alter the ratio of co- and post-transcriptional splicing in favour of the latter via CDC5L knockdown, it will be of great interest in the future to assay whether the shift from co- to post-transcriptional splicing alters alternative splicing decisions using microarrays that monitor splicing at exon–exon junctions. Identification of phosphorylated SF3b155 residues Immunoaffinity-purified, activated spliceosomes [28] (~2 pmol), were digested with trypsin, and peptide mixtures were desalted (OLIGO R3 micro-column) before phosphopeptide enrichment by Fe 3+ IMAC [47] , using Fe 3+ -loaded POROS MC20 resin (PerSeptive Biosystem). Mixtures were desalted on an OLIGO R3 precolumn (60×0.1 mm 2 ) for nano-liquid chromatography–tandem mass spectrometry analysis on a Waters Ultima Q-TOF hybrid mass spectrometer controlled by Masslynx (Waters). Proteins were identified by automated database searches using a local Mascot server v2.2 and the fragmentation patterns of the detected phosphopetides were verified by manual inspection of the corresponding mass spectometry spectra. Antibodies and cell lines Antibodies against the following human proteins were used: SC35 mouse monoclonal (BD Pharmigen, 0.5 μg μl −1 ; dilution used in IF: 1:1,000); RNA polymerase II mouse monoclonals directed against phosphorylated Ser2 (H5, Abcam, 1 μg μl −1 ) of the CTD heptad repeat (dilution used in IF: 1:1,000); RNA polymerase II RPB1 mouse monoclonals antibodies (PROGEN, cat. #65223; dilution used in IF: 1:100, western blot (WB): 1:1,000). SF3b155 mouse monoclonal antibodies raised against the MC-epitope (EQYDPFAEHRPPKIAC; stock solution: 0.5 μg μl −1 ; concentration used in WB 1:2,000; in IF 1:200); rabbit polyclonal SF3a66 (ref. 48 ), CDC5L [49] , Aly (unpublished) and hPRP8 (ref. 50 ) had a concentration of 0.5 μg μl −1 and were used at dilution of 1/1,000 for WB and 1:200 for IF. Phospho-specific SF3b155 antibodies were generated by Biogenes (Berlin, FRG) by immunizing rabbits with the following phosphopetides coupled to BSA: [C]QTPGATPKKLS (pT211), [C]RWDETPGRAK (p235), [C]SGWAETPRTDR (pT313) and [C]IGETPTPGAS (pT328) where the phosphorylated amino acid is underlined and its position indicated in parentheses. Sera were first pre-cleared by affinity selection with the respective non-phosphorylated peptides, before affinity purification with the cognate peptide. pT313-SF3b155 antibody (0.5 μg μl −1 ) was diluted at 1/1,000 for WB and 1/200 for IF. Goat anti-rabbit or anti-mouse secondary antibodies were labelled with Alexa 488, Alexa 647 or Alexa 532 (Molecular probes; 2 μg μl −1 ; dilution of 1/500 for IF). HeLa SS6 cells were obtained from ATCC. The cell line expressing H2B-GFP [34] was a kind gift of Dr Irina Solovei. In vitro splicing and blotting In vitro splicing was performed using non-radioactive pre-mRNA as previously described [51] . RNA was analysed by dot blotting using a 32 P-oligo(dT) probe [52] . Northern and western blots were performed as described [53] . Human B, B act and C complexes analysed by western blotting were affinity-purified as described previously [26] . Cell fractionation procedure HeLa cells were resuspended to ~10×10 6 per ml in HMKE buffer as described [54] to separate the cytoplasm from the nuclei. Nuclei were fractionated into chromatin and nucleoplasm fractions essentially as described previously [9] . Briefly, nuclei were resuspended in 20 mM Tris–HCl (pH 7.5), 75 mM NaCl, 0.5 mM EDTA, 50% glycerol, 2× phosphatase inhibitor (PhosStop, Roche), 2× protease inhibitor cocktail (Roche) and an equal volume of lysis buffer (10 mM HEPES-KOH (pH 7.5), 1 mM DTT, 7.5 mM MgCl 2 , 0.2 mM EDTA, 0.3 M NaCl, 0.5 M urea, 1% Triton X-100) was added. After 2×2 s vortexing, samples were incubated for 2 min on ice, and then centrifuged for 2 min, 4 °C, 16,000g, and the supernatant (soluble nucleoplasmic fraction) removed from the pellet (chromatin fraction). The latter was resuspended in buffer C (20 mM Tris–HCl (pH 7.5), 5 mM MgCl 2 , 150 mM NaCl, 1% Triton X-100, 1× phosphatase inhibitor (PhosStop, Roche), 1× protease inhibitor cocktail (Roche)), in a volume equivalent to the nucleoplasmic fraction and then sonicated in a Bioruptor (Diagenode; 30″ on, 30″ off, max intensity) in 1.5 ml microfuge tubes (300 μl per tube) for 10 min at 2 °C in a water bath. Equivalent volumes of the nucleoplasmic and chromatin fractions were subsequently used for western blotting. Glycerol gradient centrifugation and RNAse A digestion The chromatin fraction prepared as described above, was resuspended to 10×10 6 cell equivalents per ml in freshly prepared crosslink buffer (30 mM HEPES-KOH (pH 7.5), 150 mM NaCl, 2 mM EDTA, 1× PhosStop, 1× protease inhibitor cocktail, 500 μM DSP) and incubated for 1 h on ice. Crosslinking was quenched by adding Tris–HCl (pH 7.5) to a final concentration of 50 mM and incubating for 15 min. The sample was centrifuged for 10 min at 2,000 g at 4 °C and the pellet resuspended in sonication buffer (1% PEG-PEG pluronic, 0.2% Triton X-100, 30 mM Tris–HCl (pH 7.5), 3 mM EDTA, 2× phosphatase inhibitor (PhosStop, Roche), 2× protease inhibitor cocktail (Roche)). Sonication (30″ on 30″ off max intensity for 2× 30 min at 2 °C) of 300 μl of the chromatin fraction per 1.5 ml microfuge tubes. Sonicates were then layered on a 10–40% glycerol gradient containing 150 mM NaCl, 20 mM Tris–HCl, pH 7.5, and 3 mM EDTA, and centrifuged for 1 h at 60k r.p.m. in a TH660 (Thermo scientific) rotor. Gradients were fractionated into 175 μl fractions. Before SDS–polyacrylamide gel electrophoresis (PAGE), crosslinks were reversed by incubating with protein sample buffer containing 5% β-mercaptoethanol for 7 min at 100 °C. The nucleoplasmic fraction was centrifuged for 1 h at 30k r.p.m. in a TH660 rotor on identical gradients. To analyse whether the association of P-SF3b155 is RNA dependent, the chromatin fraction was incubated for 15 min at 37 °C with or without RNAse A (final concentration 1 U μl −1 ) and then microfuged at 13,000 g for 10 min. The resulting supernatant and pellet were subjected to SDS–PAGE followed by western blotting. Shearing of the chromatin fraction and immunoprecipitation The chromatin fraction was resuspended in buffer C, passed through a 27G syringe 30X, centrifuged 5 min at 16,000 g at 4 °C, and the supernatant analysed by IP. For IPs, 500 μl of nucleoplasmic or chromatin extract were diluted in 500 μl buffer C lacking Triton X-100, incubated for 4 h at 4 °C with 10 μg of antibody and then with 30 μl of protein A Sepharose for 2 h. Beads were washed 5× with buffer (20 mM Tris–HCl (pH 7.5), 5 mM MgCl 2 , 150 mM NaCl, 1% Triton X-100). RNA was recovered from the beads and analysed by northern blotting. IF microscopy and RNAi HeLa cells were grown overnight on coverslips at 37 °C in DMEM containing 10% fetal calf serum. DRB (100 μM) and SSA (100 μM) were added to the medium for 3.5 and 2 h, respectively, before analysis. For RNAi and CDC5L complementation, siRNAs and/or plasmid-encoding GFP-CDC5L (lacking 3′ UTR sequences targeted by siRNAs) were transfected into HeLa cells with lipofectamine 2000 transfection reagent (Invitrogen). siRNAs targeting CDC5L: 5′-AAGGAACTTCAACATAGATATGC-3′ (directed against the ORF) or 5′-AAGGCTGAAACTGATGTTTATCT-3′ (directed against the 3′UTR; used in complementation experiments), and Aly: 5′-CAGAGGTGGCATGACTAGAAA-3′ or 5′-CAGGAACTCTTTGCTGAATTT-3′. hPrp19/CDC5L complexes were affinity-purified as described by Grote et al . [49] and microinjected into the cytoplasm (~100 fl containing 0.7–1.3 million copies of the Prp19 complex). IF microscopy was performed as described previously [55] . Poly(A)+ FISH was performed as described [56] . The oligo(dT) probe was prepared as described [57] , using Alexa 647 (Molecular probes). Coverslips were cast in MOWIOL (Calbiochem) and analysed at 22 °C on a Zeiss LSM 510 Meta microscope equipped with Argon (488 mm), HeNe (633 nm) and solid-state (532 nm) laser sources using an oil immersion X63 APO objective with a 1.4 numerical aperture. z-stacks were acquired by setting the z-step to 150 nm and adjusting the pinhole for each fluorophore individually to obtain 500-nm thick optical slices. Image processing and analysis Deconvolution was performed with Huygens software (SVI b.v., Belgium), using a conservative SNR of 5, with a maximum of 20 iterations. All other image processing and histogram analyses were performed using ImageJ software ( http://rsb.info.nih.gov/ij ) and plots were prepared with Origin 7.5 (OriginLab). How to cite this article: Girard C. et al . Post-transcriptional spliceosomes are retained in nuclear speckles until splicing completion. Nat. Commun. 3:994 doi: 10.1038/ncomms1998 (2012).